Mechanistic insight into the interaction of BLM helicase with intra-strand G-quadruplex structures Bloom syndrome is an autosomal recessive disorder caused by mutations in the RecQ family helicase BLM that is associated with growth retardation and predisposition to cancer. BLM helicase has a high specificity for non-canonical G-quadruplex (G4) DNA structures, which are formed by G-rich DNA strands and play an important role in the maintenance of genomic integrity. Here we used single-molecule FRET to define the mechanism of interaction of BLM helicase with intra-stranded G4 structures. We show that the activity of BLM is substrate dependent, and highly regulated by a short-strand DNA (ssDNA) segment that separates the G4 motif from double-stranded DNA. We demonstrate cooperativity between the RQC and HRDC domains of BLM during binding and unfolding of the G4 structure, where the RQC domain interaction with G4 is stabilized by HRDC binding to ssDNA. We present a model that proposes a unique role for G4 structures in modulating the activity of DNA processing enzymes. G-quadruplexes (G4) are non-canonical structures formed by Hoogsteen base-pairing in guanine-rich DNA sequences [1] , [2] . There are >375,000 predicted G4 motifs in the human genome and >1,400 G4 motifs have been predicted in S. cerevisiae [3] , [4] . G4-forming sequences are found in telomeres and regulatory regions of the genome such as gene promoter regions, and can spontaneously form when single-stranded DNA (ssDNA) is generated during DNA metabolic processes [5] , [6] . The formation of G4 structures poses challenges to progression through replication, transcription and repair, and various ssDNA binding proteins and helicases are utilized for removal of G4 structures during these processes [7] , [8] , [9] , [10] , [11] , [12] , [13] . Specifically, it was previously shown that WRN, BLM, Pif1 and FANCJ helicases unwind G4 structures preferentially over duplex DNA in vitro [7] , [8] , [9] , [12] , [14] , [15] , [16] . Mutations in these helicases result in genomic instability, suggesting that their role in processing of G4 structures is central for maintaining genome integrity [17] , [18] . BLM and WRN belong to a highly conserved RecQ 3′-5′ helicase family implicated in DNA damage repair and the maintenance of genomic integrity [19] . A characteristic feature of RecQ helicases is their ability to recognize and unwind a wide variety of DNA structures. The diverse functionalities and often weak unwinding activity of RecQ family member proteins in a standard DNA helicase unwinding assay, together with their intrinsic strand-annealing activity, suggest a complex role for these enzymes that goes beyond a simple double-stranded DNA (dsDNA) unwinding function [9] . In particular, BLM and WRN have been suggested to play a role in the metabolism of G4 structures during chromosomal and telomeric replication, as well as in transcription [20] , [21] , [22] , [23] , [24] , [25] , [26] , [27] , [28] , [29] . Previous studies of the interaction of BLM with DNA substrates containing G4 structures have shown that BLM binds G4 structures with high specificity, but at the same time G4 structures can hinder BLM ssDNA translocation activity and decrease its dsDNA unwinding efficiency [30] , [31] . Here we define the interaction of BLM with G4 DNA through the use of single-molecule fluorescence resonance energy transfer (smFRET) analysis [32] , [33] . Single-molecule methods are powerful approaches capable of resolving the conformational states and dynamics of DNA and proteins in real-time that are otherwise masked by ensemble averaging. Recent single-molecule studies have provided important insights into the mechanisms of RecQ helicases with their DNA substrates and interaction of ssDNA binding proteins with G4 structures [34] , [35] , [36] , [37] . We used smFRET assays to monitor the conformational states of a human intramolecular G4 structure in the presence of BLM, and to analyze BLM unwinding of dsDNA located downstream of G4. Our data reveal that in substrates where a G4 motif is immediately adjacent to duplex DNA, BLM does not unfold the G4 motif, and is consequently unable to unwind the duplex DNA. On the other hand, introduction of a short ssDNA between the G4 motif and the duplex region restores BLM’s activity, enabling ATP-independent unfolding of the G4 structure and permitting helicase-mediated unwinding of the downstream duplex. Analysis of G4 unfolding using BLM truncation fragments suggests a specific binding configuration where unfolding of the G4 motif by the RQC domain of BLM is facilitated by binding of the HRDC domain of BLM to the ssDNA between a G4 and a duplex region. Our experiments also reveal the existence of a different BLM-mediated and ATP-dependent G4 unfolding pathway in which unfolding is assisted by external ssDNA that is homologous to the G4 sequence. These findings define a novel mechanism of interaction between BLM and G4 structures whereby the association between BLM and the G4 structure is DNA substrate selective, and results in regulation of BLM unwinding activity via the G4 folding conformation. Based on our data, we propose that intramolecular G4 sequences confer an additional level of regulation through DNA substrate selectivity and modulation of the activity of DNA metabolic enzymes (for example, helicases) in their vicinity. These sequences consequently play a pivotal role in key biological processes such as DNA replication, transcription and repair. 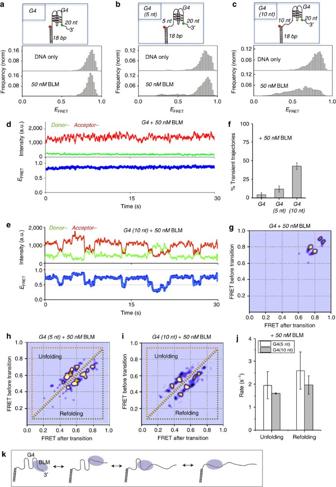Figure 1: Substrate-specific interaction of BLM with G4-forming human telomeric sequence. (a–c) BLM-mediated unfolding of G4 substrates. The illustration of each G4 DNA substrate is shown above their histograms: (a) G4 substrate, with G4 motif immediately adjacent to duplex region. No change in FRET distribution was observed following addition of 50 nM of BLM. (b) G4 (5 nt) substrate with a 5 nt ssDNA between the G4 motif and duplex region. Some change is evident upon addition of 50 nM BLM. (c) G4 (10 nt) substrate with a 10 nt ssDNA between the G4 motif and duplex region. A substantial change in the FRET distribution was detected upon addition of 50 nM BLM. Histograms were generated after subtracting the zero FRET values and truncating the photo bleached part from FRET trajectory. A minimum of 100 smFRET trajectories were used to generate the histograms. The concentration of K+was kept at 50 mM. (d) A representative single-molecule trajectory of the G4 substrate in the presence of 50 nM BLM showing persistent high FRET. Top panel: donor (green)–acceptor (red) intensities, bottom panel: corresponding FRET trajectory. (e) Representative smFRET trajectory of the G4 (10 nt) substrate in the presence of 50 nM BLM showing dynamic fluctuations in FRET signal (blue). HMM fit is in Cyan. (f) Quantification of observed transient trajectories in population percentage for each G4 substrate in the presence of 50 nM BLM. (Error bars=s.e.m.;n=5). (g–i) Generated TDP matrix for each G4 substrate in the presence of 50 nM BLM, where the colour intensity corresponds to transition probability. They-axis is the initial FRET prior to transition, and thex-axis is the final FRET after transition. (g) TDP for the G4 substrate with 50 nM BLM showing only the parallel and anti-parallel folded conformations of G4. (h,i) TDP for the G4 (5 nt) and G4 (10 nt) substrates (respectively), showing peaks corresponding to unfolding (above diagonal) and refolding (below diagonal) transitions of the G4 motif. (j) The calculated mean unfolding and refolding rates for the G4 (5 nt) and G4 (10 nt) substrates. (Error bars=s.e.m.;n>20 for all measurements). (k) Illustration of the BLM-mediated sequential unfolding–refolding transitions of the G4 substrate. DNA substrate specificity of BLM in G4 unfolding To probe the binding of BLM to G4 structures, we used a partial DNA duplex FRET substrate having a 3′-tail containing G4-forming human telomere or c-kit2 sequences (G 3 (T 2 AG 3 ) 3 and (CG 3 ) 2 CGCG(AG 3 ) 2 G, respectively, Supplementary Table 1 , sequences 2–4 and 12–15). In these FRET substrates (illustrated in Fig. 1a–c and Supplementary Fig. 1a ), the donor and acceptor dyes are placed at either end of the G4-forming sequence such that a folded G4 structure results in high FRET, while G4 unfolding would yield a low FRET signal. This arrangement enabled us to directly monitor G4 conformational changes. Previous studies have shown that monovalent cations have a pronounced effect on the stability of G4 structures; among these, K + has the highest stabilizing effect [38] . To establish a baseline for K + -dependent G4 folding in our DNA substrates, we carried out a titration of our surface-tethered FRET probe with K + and derived the population percentage of folded G4 structures from the resulting FRET histograms ( Supplementary Fig. 1b ). At low K + ion concentration, the G4 structure is predominantly unfolded ( Supplementary Fig. 1c ), whereas at 50 mM K + the G4 structure is predominantly in a folded conformation [38] . Figure 1: Substrate-specific interaction of BLM with G4-forming human telomeric sequence. ( a – c ) BLM-mediated unfolding of G4 substrates. The illustration of each G4 DNA substrate is shown above their histograms: ( a ) G4 substrate, with G4 motif immediately adjacent to duplex region. No change in FRET distribution was observed following addition of 50 nM of BLM. ( b ) G4 (5 nt) substrate with a 5 nt ssDNA between the G4 motif and duplex region. Some change is evident upon addition of 50 nM BLM. ( c ) G4 (10 nt) substrate with a 10 nt ssDNA between the G4 motif and duplex region. A substantial change in the FRET distribution was detected upon addition of 50 nM BLM. Histograms were generated after subtracting the zero FRET values and truncating the photo bleached part from FRET trajectory. A minimum of 100 smFRET trajectories were used to generate the histograms. The concentration of K + was kept at 50 mM. ( d ) A representative single-molecule trajectory of the G4 substrate in the presence of 50 nM BLM showing persistent high FRET. Top panel: donor (green)–acceptor (red) intensities, bottom panel: corresponding FRET trajectory. ( e ) Representative smFRET trajectory of the G4 (10 nt) substrate in the presence of 50 nM BLM showing dynamic fluctuations in FRET signal (blue). HMM fit is in Cyan. ( f ) Quantification of observed transient trajectories in population percentage for each G4 substrate in the presence of 50 nM BLM. (Error bars=s.e.m. ; n =5). ( g – i ) Generated TDP matrix for each G4 substrate in the presence of 50 nM BLM, where the colour intensity corresponds to transition probability. The y -axis is the initial FRET prior to transition, and the x -axis is the final FRET after transition. ( g ) TDP for the G4 substrate with 50 nM BLM showing only the parallel and anti-parallel folded conformations of G4. ( h , i ) TDP for the G4 (5 nt) and G4 (10 nt) substrates (respectively), showing peaks corresponding to unfolding (above diagonal) and refolding (below diagonal) transitions of the G4 motif. ( j ) The calculated mean unfolding and refolding rates for the G4 (5 nt) and G4 (10 nt) substrates. (Error bars=s.e.m. ; n >20 for all measurements). ( k ) Illustration of the BLM-mediated sequential unfolding–refolding transitions of the G4 substrate. Full size image To investigate the interaction of BLM with G4 DNA, surface-tethered G4 FRET substrates were incubated with 50 nM BLM in the presence of 50 mM K + . We used three different partial duplex DNA substrates, as illustrated in Fig. 1a–c and Supplementary Table 1 , with the G4 motif either immediately adjacent to the duplex region or separated by either 5 or 10 nt (substrates termed G4, G4 (5 nt) and G4 (10 nt), respectively). The histograms for these substrates before and after addition of 50 nM BLM are shown in Fig. 1a–c for telomeric G4 (upper and lower panels, respectively) and in Supplementary Fig. 2a–d for c-kit G4. Substrate G4 showed very little change in G4 folding in the presence of 50 nM BLM ( Fig. 1a and Supplementary Fig. 2a ), while substrate G4 (5 nt) displayed a change in FRET population upon addition of BLM ( Fig. 1b ). Substrate G4 (10 nt) showed a substantial change in FRET distribution upon addition of BLM, consistent with an efficient and ATP-independent unfolding of the G4 structure by BLM ( Fig. 1c and Supplementary Fig. 2b ). The unfolding of G4 structures in these substrates was found to be independent of the sequence of the ssDNA spacer used, displaying comparable unfolding for poly-dT and a mixed ssDNA spacer ( Supplementary Table 1 and Supplementary Fig. 3a,b ). To further establish that the observed unfolding of G4 structures by BLM is ATP independent, we tested the G4 unfolding activity of the helicase-dead BLM mutant (K695M; ref. 39 ). Similar to BLM, the helicase-dead BLM mutant showed no unfolding activity for the G4 substrate, but robust unfolding of the G4 (10 nt) substrate ( Supplementary Fig. 4a,b ). These findings demonstrate a unique and ATP-independent BLM–G4 substrate interaction, where BLM can efficiently unfold the G4 structure only when a ssDNA segment is present between the G4 motif and the duplex region. To determine the effect of BLM binding in these substrates, we examined the temporal behaviour of individual trajectories for each DNA substrate. Figure 1d,e displays representative smFRET trajectories from the G4 and G4 (10 nt) substrates, obtained in the presence of 50 nM BLM, where the top panels show the donor (green) and acceptor (red) intensities and the bottom panel the resulting FRET efficiencies. Trajectories from the G4 substrate ( Fig. 1d ) showed a persistent signal indicative of a stable G4 folded conformation, whereas trajectories from both the G4 (5 nt) and G4 (10 nt) substrates ( Fig. 1e and Supplementary Fig. 5 ) showed rapid fluctuations, indicative of G4 transitioning between folded and unfolded conformations. These repetitive unfolding–refolding transitions suggest that G4 unfolding by BLM is metastable such that G4 is capable of returning to its folded conformation. To determine the effect of BLM on the different substrates, we quantified the population percentage of trajectories showing fluctuations, evaluating a minimum of 300 molecules used for each substrate ( Fig. 1f ). This quantification demonstrated a clear trend, in which the percentage of trajectories exhibiting fluctuations increased with increasing distance of the G4 motif from the duplex region. A more detailed analysis of the fluctuating trajectories revealed that G4 unfolding and refolding does not switch directly from the folded to unfolded conformations (high FRET to low FRET), but occurs via intermediate states in a step-wise manner. To map the specific BLM–G4 unfolding–refolding pathways, we conducted Hidden Markov Model (HMM) analysis on the smFRET trajectories we obtained. HMM analysis is a powerful tool for analysis of single-event trajectories, and provides important characteristics of the specific states and corresponding transition probabilities [40] . The resulting HMM fit to the G4 (10 nt) trajectory was superimposed on the smFRET trajectory, and showed both a good fit and well-defined states ( Fig. 1e bottom, Cyan trace). This analysis enabled us to extract the frequency and transition rates for each FRET state and to construct a two-dimensional transition density plot (TDP). Figure 1g–i shows the TDP plots for the G4, G4 (5 nt) and G4 (10 nt) substrates, respectively, where the y -axis represents the initial FRET value before the transition and the x -axis is the final FRET value after the transition. As expected, the TDP for the G4 substrate ( Fig. 1g ) shows only two states, both at high FRET values, corresponding to the anti-parallel and parallel conformations of the G4 structures, which are the two main folded conformations of G4. The TDP for the G4 (5 nt) and G4 (10 nt) substrates shows a number of transitions starting from high FRET values down to intermediate and low FRET states, which correspond to transitions between G4 folded and unfolded states and vice-versa . Here the transitions residing below the diagonal of the TDP represent G4 refolding transitions (from lower FRET to higher FRET), whereas the transitions above the diagonal represent unfolding of the G4 structure (from higher FRET to lower FRET). The observed transition and spacing between the FRET states indicates that the G4 unfolding and refolding pathway occurs via small sequential sub-steps. This is consistent with a model in which unfolding and refolding of the four strands that participate in the G4 structure occur one strand at a time, as illustrated in the cartoon in Fig. 1k . We note that a similar observation of sequential step-wise unfolding of G4 has recently been reported for POT1-TPP1 (ref. 41 ). A comparison of the mean unfolding and refolding rates for the G4 (5 nt) and G4 (10 nt) substrates revealed that refolding rates for both substrates are higher than their unfolding rates (see Supplementary Methods for rate calculation). However, the refolding rates for the G4 (5 nt) substrate were higher than the G4 (10 nt) substrate (2.59±0.57 s −1 and 1.96±0.3 s −1 , respectively). We interpret this result to mean that BLM’s interaction and unfolding of the G4 motif in the G4 (10 nt) substrate is more stable than in the case of the G4 (5 nt) motif. This conclusion is in agreement with the overall increase in G4 unfolding efficiency in the case of the G4 (10 nt) substrate, as seen in the FRET histograms ( Fig. 1b,c ) and in the corresponding population percentage of trajectories exhibiting fluctuations ( Fig. 1f ). We ascribe the improved stability of BLM–G4 binding and unfolding efficiency in the G4 (10 nt) substrate to the placement of a longer ssDNA segment between the G4 motif and dsDNA. G4 unfolding is mediated by BLM’s RQC and HRDC domains We sought to define the specific domains of BLM that participate in G4 unfolding. The full-length BLM is a 1,417 amino acids (aa) protein, whose functional core (core BLM) is located between aa 640 and 1298, and consists of three distinct domains: the helicase core, the RecQ C-terminal (RQC) domain, and the helicase and RNaseD C-terminal (HRDC) domain [42] . While the helicase domain contains the catalytic ATP and DNA binding activities, the RQC domain and HRDC domains have been identified as being important for binding non-canonical DNA substrates including G4 (refs 39 , 42 , 43 , 44 ). We used truncated protein fragments containing the RQC and HRDC domains (RQC–HRDC: 858–1298 aa) or HRDC domain only (HRDC: 1069–1298 aa) and compared their effect on the conformations of the G4 structure in the G4 (10 nt) substrate ( Fig. 2a ). 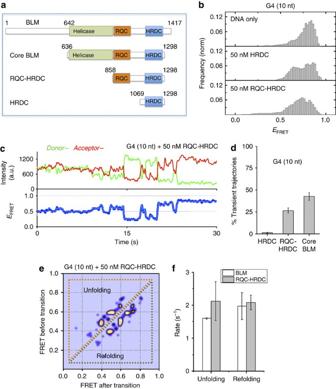Figure 2: Domain analysis of BLM–G4 unfolding activity. (a) BLM protein functional domains and truncation fragments used in this study: full-length BLM, core BLM, RQC–HRDC fragment and HRDC. (b) FRET histogram of the G4 (10 nt) substrate showing DNA only substrate (top panel), and in the presence of 50 nM HRDC fragment (mid panel) and RQC–HRDC fragment (bottom panel). (c) A representative smFRET trajectory of the G4 (10 nt) substrate in the presence of 50 nM RQC–HRDC fragment, showing rapid FRET fluctuations (blue curve). HMM fit is in cyan. (d) Quantification of population percentage of transient trajectories for the G4 (10 nt) substrate in the presence of 50 nM of HRDC and RQC–HRDC fragments and core BLM. (Error bar=s.e.m.;n=4). (e) TDP for the G4 (10 nt) substrate in the presence of 50 nM RQC–HRDC fragment. (f) Quantification of the mean unfolding and refolding rates for the G4 motif of the G4 (10 nt) substrate, in the presence of 50 nM RQC–HRDC fragment or core BLM. (Error bar=s.e.m.;n>24 for all measurements). Figure 2b shows the resulting smFRET histograms for the G4 (10 nt) substrate in the presence of 50 nM HRDC or 50 nM RQC–HRDC (mid and bottom panels, respectively). Both fragments resulted in altered smFRET histograms, as compared with the G4 (10 nt) DNA only histogram (top panel). However, while the HRDC fragment resulted in a change in FRET populations within the G4 folded conformation, the RQC–HRDC fragment resulted in a broader distribution corresponding to unfolded conformations of G4. Analysis of individual smFRET trajectories for each of the fragments revealed that the RQC–HRDC fragment resulted in trajectories undergoing rapid fluctuations ( Fig. 2c ) similar to the dynamics observed for BLM, indicative of unfolding and refolding dynamics, whereas the HRDC fragment displayed a uniform and stable signal corresponding to a folded G4 conformation. Figure 2d shows a quantification of the population percentage of fluctuating trajectories for each fragment, where both BLM and RQC–HRDC showed a considerable number of fluctuating trajectories, while HRDC did not ( Supplementary Fig. 6a,b ). The characteristic behaviour observed for trajectories with the RQC–HRDC fragment revealed transitions between discrete steps, similar to those seen with BLM. We applied HMM analysis to obtain the states and corresponding rates for the observed transitions, and determined how these compared with the metrics obtained for BLM. The resulting TDP for the G4 (10 nt) substrate in the presence of 50 nM RQC–HRDC shows discrete transitions corresponding to sequential sub-steps of unfolding and refolding of G4 ( Fig. 2e ). We note that these transitions are comparable to the transitions observed for the same substrate in the presence of BLM. We next quantified the G4 unfolding and refolding rates for RQC–HRDC, and compared them with the rates obtained for BLM ( Fig. 2f ). While the G4 refolding rates for both BLM and RQC–HRDC were found to be similar (1.96±0.3 s −1 and 2.08±0.1 s −1 , respectively), the unfolding rate of RQC–HRDC was higher than the unfolding rate of BLM (2.12±0.4 s −1 and 1.5±0.01 s −1 , respectively), possibly due to an enhanced overall stability of BLM binding to DNA, as compared with RQC–HRDC [42] . We infer from the observation that both HRDC and RQC–HRDC bind the G4 substrate, while only RQC–HRDC can efficiently unfold it, that the HRDC domain assists in stabilizing the RQC domain interaction with G4, possibly by binding to the ssDNA segment downstream of G4. Figure 2: Domain analysis of BLM–G4 unfolding activity. ( a ) BLM protein functional domains and truncation fragments used in this study: full-length BLM, core BLM, RQC–HRDC fragment and HRDC. ( b ) FRET histogram of the G4 (10 nt) substrate showing DNA only substrate (top panel), and in the presence of 50 nM HRDC fragment (mid panel) and RQC–HRDC fragment (bottom panel). ( c ) A representative smFRET trajectory of the G4 (10 nt) substrate in the presence of 50 nM RQC–HRDC fragment, showing rapid FRET fluctuations (blue curve). HMM fit is in cyan. ( d ) Quantification of population percentage of transient trajectories for the G4 (10 nt) substrate in the presence of 50 nM of HRDC and RQC–HRDC fragments and core BLM. (Error bar=s.e.m. ; n =4). ( e ) TDP for the G4 (10 nt) substrate in the presence of 50 nM RQC–HRDC fragment. ( f ) Quantification of the mean unfolding and refolding rates for the G4 motif of the G4 (10 nt) substrate, in the presence of 50 nM RQC–HRDC fragment or core BLM. (Error bar=s.e.m. ; n >24 for all measurements). Full size image To further test the hypothesis that the observed ATP-independent unfolding of G4 is unique and mediated by RQC–HRDC domains, we tested whether G4 disruption in these substrates can be carried out by other DNA helicases. We used two RecQ family helicases, WRN and RecQL5: WRN has RQC and HRDC domains similar to BLM, while RecQL5 has an RQC domain but no HRDC domain [27] . As with BLM, WRN was able to unfold the G4 structure in the G4 (10 nt) substrate, but not in the G4 substrate alone ( Supplementary Fig. 7a,b ); on the other hand, RecQL5 did not display any G4 unfolding activity with either of these substrates ( Supplementary Fig. 7c ). We also tested the Pif1 5′–3′ helicase, previously shown to have robust G4 unwinding activity and to be implicated in the metabolism of G4 structures [10] , [17] , [45] , [46] . In a recent smFRET study, Pif1 was shown to bind at the 3′-tailed DNA junction, reeling in the 3′-ssDNA tail to unfold intramolecular G4 structures in an ATP-dependent manner [46] . In agreement with that study, we found that the binding of Pif1 did not result in unfolding of the G4 structure in either substrate ( Supplementary Fig. 7d ). These results indicate that ATP-independent G4 unfolding is carried by HRDC–RQC domains and that this is a function that is unique to RecQ helicases. G4 structure regulates activity of BLM at proximal dsDNA We sought to determine whether BLM’s substrate selectivity in unfolding the G4 motif also affects its unwinding activity of a duplex located downstream of the G4 motif. Recent studies have shown that G4 inhibits the ssDNA translocation activity of BLM and reduces the overall efficiency of BLM-mediated duplex unwinding [31] . We first tested the regular G4 substrate (that is, having no ssDNA between the G4 and duplex region); this showed no G4 unfolding upon addition of BLM. Full unwinding of the duplex part in these FRET substrates will result in a complete loss of the donor (Cy3) labelled DNA strand and consequently loss of the fluorescence signal [32] . For our unwinding assay, BLM and ATP were added to the perfusion chamber containing surface-tethered DNA FRET substrates and incubated for 2 min, followed by a wash with high salt (500 mM NaCl) buffer to terminate the reaction. To quantify the unwinding yield, surface-tethered FRET molecules were counted before and after the unwinding reaction. 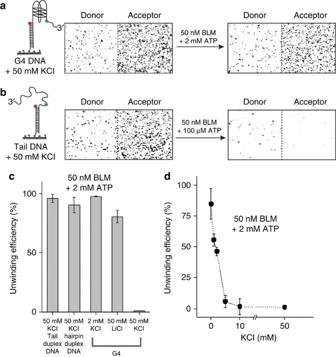Figure 3: Regulation of BLM unwinding activity by G4 folding. (a,b) Left—cartoon of the substrates used. Right—images of individual DNA substrate molecules before and after the unwinding reaction, where donor molecules are shown at the left and corresponding acceptor molecules are at the right. Unwinding was not seen for the G4 substrate (a), whereas complete unwinding was seen for the regular tailed duplex substrate (b). (c) Quantification of BLM unwinding efficiency at 50 nM BLM and 2 mM ATP for the G4 substrate at various buffer conditions. (i) Regular tailed duplex (b) in the presence of 50 mM KCl. (ii) hairpin substrate (Supplementary Fig. 1A) in the presence of 50 mM KCl. (iii–v) G4 substrate in the presence of: (iii) 2 mM KCl; (iv) 50 mM LiCl and (v) 50 mM KCl. (Error bar=s.e.m.;n=4). (d) BLM unwinding activity of the G4 substrate as a function of KCl concentration (Error bar=s.e.m.;n=5). Figure 3a,b shows images of individual FRET molecules obtained before and after the unwinding reaction with G4 DNA substrate ( Fig. 3a ) and regular partial duplex DNA substrate ( Fig. 3b ), where both substrates contain a duplex region of the same length and sequence (see Supplementary Table 1 ). These images clearly show that BLM is unable to unwind the G4 substrates, which persist after the unwinding reaction, whereas the majority of partial duplex DNA molecules were unwound and removed from the surface even in the presence of 50 nM BLM and 100 μM ATP. Figure 3: Regulation of BLM unwinding activity by G4 folding. ( a , b ) Left—cartoon of the substrates used. Right—images of individual DNA substrate molecules before and after the unwinding reaction, where donor molecules are shown at the left and corresponding acceptor molecules are at the right. Unwinding was not seen for the G4 substrate ( a ), whereas complete unwinding was seen for the regular tailed duplex substrate ( b ). ( c ) Quantification of BLM unwinding efficiency at 50 nM BLM and 2 mM ATP for the G4 substrate at various buffer conditions. (i) Regular tailed duplex ( b ) in the presence of 50 mM KCl. (ii) hairpin substrate ( Supplementary Fig. 1A ) in the presence of 50 mM KCl. (iii–v) G4 substrate in the presence of: (iii) 2 mM KCl; (iv) 50 mM LiCl and (v) 50 mM KCl. (Error bar=s.e.m. ; n =4). ( d ) BLM unwinding activity of the G4 substrate as a function of KCl concentration (Error bar=s.e.m. ; n =5). Full size image To establish that the observed low yield of unwinding is indeed due to formation of G4 structures, we carried out two additional unwinding experiments with the G4 substrate, but under buffer conditions where a G4 structure cannot readily form. Instead of 50 mM KCl, we used either 2 mM KCl, where the G4 structure is predominantly in its unfolded state, or 50 mM LiCl, as Li + does not stabilize G4 structures [47] . Under these conditions, BLM showed a comparable unwinding efficiency to that observed on the regular partial duplex DNA substrate ( Fig. 3c ), confirming that G4 structure formation indeed inhibits BLM-mediated unwinding of dsDNA when it is positioned downstream. To confirm that inhibition of unwinding is specific for the G4 containing substrate, rather than universal for substrates containing secondary structures, we used a hairpin substrate having a high GC base content ( T m ~50 °C) with approximately the same length of G4 region ( Supplementary Table 1 and Supplementary Fig. 1a ). We found that unwinding of the hairpin substrate by BLM under the same buffer conditions used for the G4 substrate was highly efficient ( Fig. 3c ), confirming that the G4 structure specifically inhibits BLM unwinding. To further establish the effect of G4 folding on BLM unwinding activity in the G4 substrate, we quantified BLM’s unwinding yield as a function of KCl concentration ( Fig. 3d ). This experiment showed that the unwinding yield steeply decreased with increasing KCl concentration and is fully inhibited at ~10 mM KCl and higher. The KCl-dependent reduction in unwinding yield correlates well with the increase in G4 folding stability at those concentrations ( Supplementary Fig. 1b ). Next, we characterized BLM’s unwinding activity for the G4 (5 nt) and G4 (10 nt) substrates, which showed elevated unfolding of G4 structures by BLM as compared with regular G4 substrate containing no ssDNA spacer ( Fig. 1 ). Quantification of the BLM unwinding yield for these substrates and a regular G4 substrate is plotted in Fig. 4a and Supplementary Fig. 8a,b ; the data show that BLM can efficiently unwind these substrates compared with the G4 substrate. Substrate G4 (10 nt) had a higher unwinding efficiency than G4 (5 nt), suggesting that initial unfolding of the G4 structure determines BLM’s ability to unwind the downstream duplex. To rule out the possibility that BLM initiates unwinding of the downstream duplex directly from the 10 nt ssDNA, we used a gapped-tailed substrate ( Supplementary Fig. 9 and Supplementary Table 1 ), which showed low unwinding efficiency compared with the G4 (10 nt) substrate. This observation confirms that unwinding is not initiated from the 10 nt ssDNA segment, but occurs after BLM unfolds and passes the G4 motif. We note that the reduced unwinding efficiency we observe for the gapped substrate is consistent with previous reports, and stem from BLM’s substrate affinity rather than its binding footprint [48] . To further establish the correlation between substrate-dependent G4 unfolding and the unwinding of downstream duplex, we tested the unwinding activity of WRN and RECQL5 in these substrates. Consistent with the ATP-independent G4 unfolding observed for these helicases ( Supplementary Fig. 7a,b ), WRN was able to unwind the G4 (10) but not the G4 substrate, whereas REQCL5 was unable to unwind either substrate ( Supplementary Fig. 10 ). We conclude that the RQC–HRDC-mediated unfolding of the G4 structure in these substrates governs the ability of the helicase to unwind downstream dsDNA. 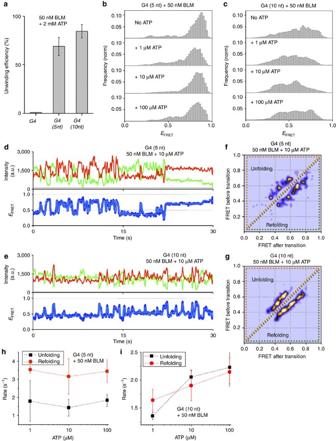Figure 4: BLM-dependent unwinding activity on a G4 substrate. (a) Quantification of BLM unwinding efficiency at 50 nM BLM and 2 mM ATP for the G4, G4 (5 nt) and G4 (10 nt) substrates (Error bar=s.e.m.;n=5). (b,c) FRET histograms of the G4 (5 nt) and G4 (10 nt) substrates (b,c, respectively) in the presence of 50 nM BLM and at different ATP concentrations. (d,e) Representative single-molecule trajectories of the G4 (5 nt) and G4 (10 nt) substrates (d,e, respectively) in the presence of 50 nM BLM and 10 μM ATP. FRET trajectories were fitted with HMM (Cyan). (f,g) Generated TDP matrix of the G4 (5 nt) and G4 (10 nt) substrates (f,g, respectively) in the presence of 50 nM BLM and 10 μM ATP. (h,i) The calculated mean unfolding and refolding rates for the G4 (5 nt) and G4 (10 nt) substrates (h,i, respectively) in the presence of 50 nM BLM and at different ATP concentrations. (Error bars=s.e.m.;n>15 for all measurements). Figure 4: BLM-dependent unwinding activity on a G4 substrate. ( a ) Quantification of BLM unwinding efficiency at 50 nM BLM and 2 mM ATP for the G4, G4 (5 nt) and G4 (10 nt) substrates (Error bar=s.e.m. ; n =5). ( b , c ) FRET histograms of the G4 (5 nt) and G4 (10 nt) substrates ( b , c , respectively) in the presence of 50 nM BLM and at different ATP concentrations. ( d , e ) Representative single-molecule trajectories of the G4 (5 nt) and G4 (10 nt) substrates ( d , e , respectively) in the presence of 50 nM BLM and 10 μM ATP. FRET trajectories were fitted with HMM (Cyan). ( f , g ) Generated TDP matrix of the G4 (5 nt) and G4 (10 nt) substrates ( f , g , respectively) in the presence of 50 nM BLM and 10 μM ATP. ( h , i ) The calculated mean unfolding and refolding rates for the G4 (5 nt) and G4 (10 nt) substrates ( h , i , respectively) in the presence of 50 nM BLM and at different ATP concentrations. (Error bars=s.e.m. ; n >15 for all measurements). Full size image To determine how ATP affects BLM’s G4 unfolding activity in these substrates, we added BLM together with ATP, and then monitored G4 FRET efficiency as a function of ATP concentration. We used ATP concentrations of 1, 10 and 100 μM because at these concentrations unwinding of the downstream duplex does not dominate the observed dynamics; thus the G4 refolding–unfolding transition can be extracted and analyzed ( Fig. 4b,c ). While both substrates displayed a change in the FRET distribution upon addition of ATP, the G4 (10 nt) substrate showed the most substantial redistribution of the FRET populations with ATP. Analysis of individual trajectories for the two substrates showed rapid unfolding–refolding transitions for the G4 (5 nt) and G4 (10 nt) substrates, respectively ( Fig. 4d,e ). These fluctuations are more dynamic than the fluctuations observed for BLM unfolding–refolding transitions in the absence of ATP; this may be due to BLM’s ATP-dependent translocation dynamics away from the G4 region. To obtain the specific transition states and the refolding and unfolding rates as a function of ATP, we carried out HMM analysis on individual trajectories from each substrate and generated TDP images. Figure 4f,g shows the TDP for G4 (5 nt) and G4 (10 nt) substrates in the presence of 50 nM BLM and 10 μM ATP. The TDP for the G4 (10 nt) substrate showed broadening of the transition peaks, whereas transitions for the G4 (5 nt) substrate formed defined peaks (see also Supplementary Fig. 11a–d ). To determine whether the TDP reflects a specific ATP-induced G4 folding response, we plotted the unfolding and refolding rates for each substrate as a function of [ATP] for both G4 (5 nt) and G4 (10 nt) substrates ( Fig. 4h,i , respectively). While the unfolding and refolding rates for the G4 (5 nt) substrate were largely unchanged as a function of [ATP], the rates for the G4 (10 nt) substrates followed a clear trend of increase with increasing ATP concentration. The increase in both unfolding and refolding rates with ATP is indicative of BLM translocating through the G4 region following G4 unfolding, which would result in an increase in both unfolding (into the G4 structure) and refolding (away from G4 towards the duplex region). The fact that this dependence is not observed for the G4 (5 nt) substrate are consistent with the dependence of this behaviour on the availability of the longer ssDNA segment between G4 and the duplex. Specifically, the length of the ssDNA spacer will govern both G4 unfolding efficiency and consequently initiation of helicase activity, so that unwinding is observed on G4 substrates where the G4 is efficiently unfolded by BLM and enough ssDNA is produced. In this event, the observed inhibition of unwinding can be ascribed to steric occlusion induced by G4 folding. G4 complementary strand assists downstream duplex unwinding We next sought to determine whether BLM’s unwinding activity in the G4 substrate could be restored via external disruption of G4 folding. To do this, we used either replication protein A (RPA) or a short ssDNA complementary to the G4 sequence; these were added at various concentrations along with BLM (50 nM) and ATP (2 mM). Contrary to our expectations, RPA (1 or 10 nM) did not assist core BLM unwinding of the G4 substrate either when added together with BLM and ATP, or when pre-incubated with the DNA substrate prior to addition of BLM and ATP. Since core BLM lacks the RPA interaction domain [49] , we also carried out these experiments with full-length BLM, which, in a similar manner to core BLM, did not show enhanced unwinding in the presence of RPA ( Supplementary Fig. 12a ). In contrast, addition of the complementary strand (CS) along with BLM and ATP resulted in efficient unwinding of the downstream duplex. 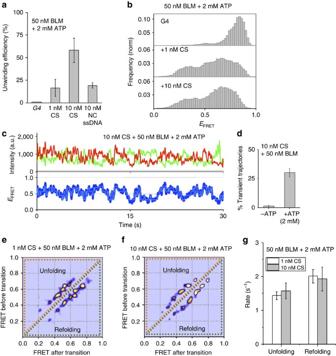Figure 5: G4 complementary strand-assisted unwinding of the G4 substrate. (a) Quantification of BLM unwinding efficiency at 50 nM BLM and 2 mM ATP for the G4 substrate in the presence of no CS, 1 nM CS or 10 nM CS, or 10 nM not complementary (NC) ssDNA (Error bar=s.e.m.;n=5). (b) FRET histograms of the G4 substrate in the presence of 50 nM BLM and 2 mM ATP with either no CS (top panel), 1 nM CS (mid panel) or 10 nM CS (bottom panel). (c) Representative single-molecule trajectories of the G4 substrate in the presence of 50 nM BLM, 2 mM ATP and 10 nM CS. FRET trajectories were fitted with HMM (Cyan). (d) Quantification of population percentage of transient trajectories for the G4 substrate in the presence of 50 nM BLM and 10 nM CS and with our without 2 mM ATP. (Error bar=s.e.m.;n=4). (e,f) Generated TDP matrix of the G4 substrate in the presence of 50 nM BLM and 2 mM ATP as well as either 1 nM CS or 10 nM CS (d,e, respectively). (g) The calculated mean unfolding and refolding rates for the G4 substrate in the presence of 50 nM BLM, 2 mM ATP and at 1 nM or 10 nM CS concentration. (Error bars=s.e.m.;n>34 for all measurements). Figure 5a shows the unwinding yield of the G4 substrate by 50 nM BLM and 2 mM ATP either added alone or in the presence of 1 or 10 nM CS, where the addition of CS enabled BLM to unwind the downstream duplex, and the unwinding efficiency increased with increasing CS concentration. To determine whether the external ssDNA-assisted G4 disruption and unwinding is homology dependent, we measured the unwinding of G4 substrate in the presence of ssDNA of similar length to CS, but with a sequence that was not complementary to G4. This resulted in a considerably lower unwinding efficiency ( Fig. 5a ), demonstrating that the external ssDNA-assisted unwinding of the G4 substrate is homology dependent. Figure 5b shows the resulting smFRET histograms for each concentration of CS compared with no CS, where a substantial shift and redistribution of FRET values is seen for both 1 and 10 nM CS. Figure 5c shows a representative smFRET trajectory of the G4 substrate in the presence of 10 nM CS, 50 nM BLM and 2 mM ATP: here the data reveal a display of dynamic fluctuations, representing rapid unfolding and refolding transitions. These dynamics are in contrast to the stable FRET trajectory obtained for the G4 substrate in the presence of 50 nM BLM and 2 mM ATP, when no CS was added ( Supplementary Fig. 12b ). To determine the role of ATP in G4 unfolding, we quantified the number of trajectories showing fluctuations in the presence and absence of ATP ( Fig. 5d ). In contrast to the ATP-independent unfolding in the G4 (5 nt) and G4 (10 nt) substrates, unfolding–refolding transitions were not observed in the absence of ATP, confirming that CS-assisted G4 unfolding is ATP dependent. To characterize the observed transitions, we carried out HMM analysis of trajectories at two concentrations of CS, and generated their TDP ( Fig. 5e,f ). The resulting TDP for both CS concentrations showed similar transition probabilities. This verifies that the occurrence of G4 unfolding, but not the unfolding pathway itself, depends upon CS concentration. Moreover, this finding suggests that CS-assisted unwinding is mediated by a single CS per G4 substrate. This conclusion is further supported by the unfolding–refolding rates ( Fig. 5g ), which remained unchanged with increased concentration of CS. Figure 5: G4 complementary strand-assisted unwinding of the G4 substrate. ( a ) Quantification of BLM unwinding efficiency at 50 nM BLM and 2 mM ATP for the G4 substrate in the presence of no CS, 1 nM CS or 10 nM CS, or 10 nM not complementary (NC) ssDNA (Error bar=s.e.m. ; n =5). ( b ) FRET histograms of the G4 substrate in the presence of 50 nM BLM and 2 mM ATP with either no CS (top panel), 1 nM CS (mid panel) or 10 nM CS (bottom panel). ( c ) Representative single-molecule trajectories of the G4 substrate in the presence of 50 nM BLM, 2 mM ATP and 10 nM CS. FRET trajectories were fitted with HMM (Cyan). ( d ) Quantification of population percentage of transient trajectories for the G4 substrate in the presence of 50 nM BLM and 10 nM CS and with our without 2 mM ATP. (Error bar=s.e.m. ; n =4). ( e , f ) Generated TDP matrix of the G4 substrate in the presence of 50 nM BLM and 2 mM ATP as well as either 1 nM CS or 10 nM CS ( d , e , respectively). ( g ) The calculated mean unfolding and refolding rates for the G4 substrate in the presence of 50 nM BLM, 2 mM ATP and at 1 nM or 10 nM CS concentration. (Error bars=s.e.m. ; n >34 for all measurements). Full size image We note that when CS was added to the G4 substrate alone no change was observed in the G4 conformation, confirming that the CS interaction with G4 is not random and is facilitated by BLM ( Supplementary Fig. 12c ). While BLM has strand-annealing activity, this interaction is not carried out via its annealing activity, as the core BLM lacks the domain for this activity [50] . This was also verified by testing CS-assisted unwinding of the G4 substrate using full-length BLM, which did not result in an increase in unwinding yield as compared with the core BLM ( Supplementary Fig. 12d ). We conclude that the HRDC domain may play a role here as well, in which the helicase core and the RQC domain are in contact with the G4 substrate, while the HRDC domain captures the CS and facilitates the destabilization of G4 and unwinding of the downstream duplex. Using smFRET we show that BLM requires a ssDNA segment between the G4 motif and duplex region to efficiently unfold intramolecular G4 DNA structures. The unfolding of G4 is ATP independent, is mediated by the RQC and HRDC domains, and occurs in a sequential manner, where G4 does not transition directly to the unfolded conformation, but proceeds via sub-steps. Moreover, BLM unfolding of G4 is metastable, which allows for repetitive refolding and unfolding transitions to occur. The length of ssDNA segment determines the magnitude of G4 destabilization and consequently unwinding of a downstream duplex. Taken together, our observations demonstrate that the BLM–G4 interaction constitutes a unique substrate-dependent activity. Based on our findings, we propose an integrated model for the cooperative binding and interaction of BLM with an intramolecular G4 structure ( Fig. 6 ). Unfolding of G4 by BLM is mediated via cooperative binding of the RQC and HRDC domains, where the RQC interaction with G4 is stabilized by HRDC binding to the ssDNA segment between G4 and the duplex ( Fig. 6a ). In addition, the ssDNA binding activity of the HRDC domain may also play a role in capturing the CS to promote BLM’s CS-assisted unwinding of the regular G4 substrate, as illustrated in Fig. 6b . Previous studies have identified the RQC domain as having a high affinity for G4 structures, whereas the HRDC domain was shown to play a regulatory role in HJ dissolution and binding to ssDNA [39] , [43] , [44] , [51] . Recent structure-based studies have suggested a model for BLM HJ interaction, in which HRDC binds ssDNA at the junctions and operates at a distance from the RQC and helicase core [52] , [53] . This distant interaction is afforded by a long flexible linker (13 aa~10 nm) between the RQC and HRDC, which is sufficient for binding ssDNA over the folded G4 structure (~5 nm) [52] . Cooperative binding at a distance may explain helicase selectivity in unfolding and processing specific G4 substrates. 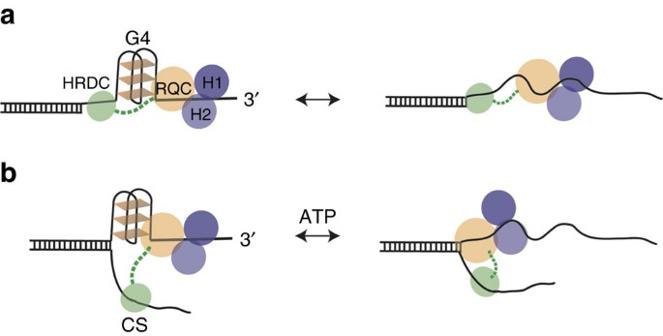Figure 6: Proposed model for BLM–G4 substrate selectivity, unfolding of a G4 motif and regulation of BLM activity via binding cooperativity of RQC–HRDC domains. (a) In binding to substrates containing ssDNA between G4 and duplex DNA, the HRDC domain, via its flexible linker, binds the ssDNA between G4 and the duplex region thus anchoring and stabilizing RQC interaction with G4, facilitating its unfolding. (b) ATP-dependent complementary strand-assisted unfolding of G4, the HRDC binds CS assisting to destabilize G4 structure. Figure 6: Proposed model for BLM–G4 substrate selectivity, unfolding of a G4 motif and regulation of BLM activity via binding cooperativity of RQC–HRDC domains. ( a ) In binding to substrates containing ssDNA between G4 and duplex DNA, the HRDC domain, via its flexible linker, binds the ssDNA between G4 and the duplex region thus anchoring and stabilizing RQC interaction with G4, facilitating its unfolding. ( b ) ATP-dependent complementary strand-assisted unfolding of G4, the HRDC binds CS assisting to destabilize G4 structure. Full size image There is a growing body of evidence that G4 structures and G4-associated proteins play a central role in chromosome metabolism. Several hundred thousand DNA sequences with the potential to form intra-stranded G4 structures are present in the human genome [5] , [6] , [54] , [55] . These sequences will spontaneously form intra-stranded G4 structures when ssDNA is generated during DNA replication, transcription and repair, and if not removed will obstruct these processes [18] , [56] . Several human helicases have been implicated in the removal of G4 structures, including FANCJ, RTEL1 and Pif1 (having a 5′–3′ directionality), and two RecQ family helicases, BLM and WRN (each with a 3′–5′ directionality) [57] . Importantly, among the five human RecQ family helicases, only BLM and WRN have both RQC and HRDC domains [27] . With respect to their function in the removal of G4 structures, BLM and WRN have been found to associate with the replication machinery in both chromosomal and telomere replication [20] , [22] , [23] , [24] , [25] , [26] , [35] , [58] . During replication, intramolecular G4 structures can form after dsDNA unwinding by the replicative helicase and impede leading or lagging strand synthesis, resulting in an accumulation of ssDNA and the collapse of the replication fork. Based on our findings and proposed model, BLM and WRN may assist in the removal of characteristic replication fork G4 structures, as previously suggested [19] . In addition, the substrate selectivity and removal of G4 structures by BLM and WRN may play an important role during transcription. Recent studies have identified a novel correlation between the presence of G4-forming sequences in the regulatory regions of genes and the regulation of gene expression by BLM and WRN helicases [28] , [59] . The regulation of gene expression by BLM and WRN may thus be mediated by removal of G4 structures formed on ssDNA within the transcription R-loop, which would otherwise impede gene expression. In a recent smFRET study of Pif1 helicase it was shown that the removal of G4 structures is ATP dependent and mediated by reeling of a ssDNA tail [46] . Importantly, this study found that the binding of Pif1 and reeling of ssDNA is only permitted in substrates having a ssDNA spacer between the dsDNA and G4. While the underlining mechanisms for G4 removal by Pif1 and BLM are distinct, the striking similarity in the requirement for a ssDNA spacer suggests a unique DNA substrate selectivity among G4 specific helicases. Such selectivity may be jointly utilized in G4 metabolism. For example, BLM has been shown to interact with FANCJ, a helicase-like BLM implicated in DNA repair but with opposite directionality [60] . FANCJ has been shown to unwind G4 structures in a unique manner compared with representative Fe-S cluster helicases [61] , and has been implicated with BLM in a common pathway that maintains epigenetic stability at G4 DNA [62] . We predict that G4 structural selectivity and cooperation among other DNA processing enzymes provides an additional level of functional regulation that plays a critical role in genomic metabolism. DNA preparations All oligonucleotides ( Supplementary Table 1 ) were purchased from Integrated DNA Technology (IDT). For annealing, the appropriate oligonucleotides were mixed and heated for 3 min at 94 °C followed by slow cooling. Protein purification To investigate the interaction of BLM with G4 DNA, we used the core BLM helicase, a truncated BLM variant (BLM 636–1298 ) containing RQC and HRDC domains that retain the unwinding and translocation activity of the wild-type BLM [30] , [36] , [42] . In addition, we used core WRN (418–1,232) containing the RQC and HRDC domains, human Pif1 helicase domain (206–641) shown to binding G4 structures and unwind inter-stranded G4, helicase-dead core BLM (K695M) and RecQL5. Full-length BLM was used to verify our observations relating to core BLM. Core BLM (aa 636–1,298) was expressed in Escherichia coli system and purified using tag affinity capture [63] . After cleavage with TEV protease, the protein retains the vector-derived sequences SM and ENLYFQ at the N- and C-termini, respectively. Truncated fragments (RQC–HRDC: aa 858–1,298 and HRDC: aa 1,069–1,298) were cloned into vector pNIC28-Bsa4 and purified on HisTrap FF and Superdex 75 columns [64] ; the proteins were used without removal of the N-terminal His 6 tags. Al purified proteins maintained their native state as determined by their gel filtration absorption profile, which migrates as a single symmetrical peak ( Supplementary Fig. 13 for RQC–HRDC fragment). Core WRN, Pif1 HD were expressed and purified from a Baculovirus expression vector system [65] , [66] . For expression and purification RecQL5 and helicase-dead core BLM we used E. coli expression system and purified using an affinity tag [42] , [67] . Expression and purification of the recombinant full-length BLM protein was performed using a three-step protocol [68] : nickel affinity, heparin affinity and gel filtration chromatography. In brief, yeast cell pellets expressing human BLM (JEL1+pJK1_BLM) were re-suspended in an equal volume of lysis buffer, consisting of 50 mM Hepes-KOH pH 7.4, 1 M KCl, 1 mM DTT, 10% glycerol, 1 mM PMSF and supplemented with complete EDTA-free protease inhibitor (Roche). Benzonase (E1014-25kU, Sigma) was added at 25 U ml −1 . An equal volume of glass beads (425–600 μm, Sigma) was added to the suspension and the cells were lysed by vigorous shaking for 10 × 1 min with incubations of 30 s on ice after each burst. The lysate was clarified at 350,000 g for 1 h at 4 °C. The supernatant was adjusted to contain 15 mM imidazole, filtered through 45 μm filter and loaded onto HisTrap column (GE Healthcare). The column was washed with lysis buffer containing 15 mM imidazole. Subsequently, the washing buffer was exchanged to the same buffer with reduced salt concentration (500 mM KCl instead of 1 M). Several step gradients of this buffer, containing different concentrations up to 80 mM imidazole, were used further to wash the column. The column was eluted using a 10-column volume gradient between 80 and 500 mM imidazole. Eluted fractions containing BLM were pooled, diluted to adjust the final pH and KCl concentration to 7.5 and 125 mM, respectively, and were loaded onto a Heparin column (GE Healthcare). The column was washed with a buffer containing 50 mM Hepes-KOH pH 6.8, 125 mM KCl, 1 mM DTT, 10% glycerol and supplemented with complete EDTA-free protease inhibitor. The BLM protein was eluted using a 20-column volume gradient between 150 mM and 1 M KCl. Eluted fractions containing the BLM protein were pooled and concentrated up to 10-fold using an Amicon Ultra-4 cetrifugal filter device (50 K cut-off, Millipore). The pooled eluate was loaded onto a gel filtration column (Superose 6 10/300 GL; GE Healthcare) using a buffer containing 50 mM Hepes-KOH pH 7.4, 10% glycerol, 500 mM KCl and 1 mM DTT. Fractions containing recombinant BLM, as determined by Coomassie-stained SDS–PAGE, were pooled and the protein was dialyzed against a buffer containing 50 mM Hepes-KOH pH 7.2, 250 mM KCl, 10% glycerol and 1 mM DTT. Finally, the protein was stored at −80 °C in small aliquots. Single-molecule fluorescence resonance energy transfer Reactions were carried out at room temperature in a standard buffer composed of 50 mM Tris-HCl (pH 8.0), 2 mM MgCl 2 and an oxygen scavenging system (1 mg ml −1 glucose oxidase, 0.4% (w/v) D-glucose, 0.02 mg ml −1 catalase and 2 mM Trolox) [32] . The concentration of K + in the buffer was varied and is indicated accordingly in the text or in the figure legends. All experiments had 100 pM DNA immobilized on a PEG-coated quartz surface with biotin–neutravidin linkage. Microscopy set-up and single-molecule analysis We used a custom-built microscopy set-up based on a Leica DMI3000 microscope equipped with an HCX PL APO × 63 numerical aperture=1.47 OIL CORR TIRF objective followed by achromatic × 2 tube lens magnification. The microscope was coupled to 532 and 640 nm solid-state lasers to excite the sample at Total-Internal-Reflection illumination mode for improved signal to noise ratio and reject out plane fluorescence. Sample emission was collected and split into two channels through the use of proper dichroic and emission narrow-band bandpass filters (filter for green channel 580/60, filter for red channel 680/40, Semrock) in conjunction with the use of a Dual View (DV2-Photometrics) to image two colours simultaneously, side-by-side, onto a single EM-CCD camera (Andor iXon+ 897) acquiring at 33 Hz. For accurate alignment and mapping of the two colour channels, we first imaged diffraction-limited fluorescent beads that have wide emission spectra spanning both channels (Invitrogen). The location of the beads was matched for both channels, and a mapping matrix was generated using an IDL (Exelis Visual Information Solutions) custom mapping routine. Briefly, this routine is based on the use of a polynomial morph-type mapping function, whereby mapping coefficients are generated by Gaussian and centroid fits to the sub-diffraction limit point-spread functions of the fluorescence beads. Another IDL code was used, along with the mapping matrix, to extract corresponding single-molecule donor and acceptor spots into single-molecule trajectories. Programmes written in MATLAB were used to view and analyze single-molecule fluorescence time trajectories. FRET efficiency, E FRET , was approximated as the ratio between the acceptor intensity and the sum of acceptor and donor intensities. Each smFRET histogram was generated by a minimum of a 100 trajectories, and the contribution of each trajectory was normalized in the histogram so that the weight of the FRET states from each molecule in the histogram will be identical. For unwinding yield quantification, dual images were analyzed using a threshold and cluster counting routine, to obtain the number of molecules observed in the field of view. HMM analysis, TDP and derived statistics were done using freely available HMM and TDP software (Ha lab) [40] . The resulting TDP plots showed a number of symmetrical peaks for folding and refolding transitions, along with a low intensity singular peak for refolding into higher FRET state. We interpret this peak as possible ssDNA looping mediated by the HRDC domain occurring after unfolding of the G4 structure. To generate the mean rates for folding (unfolding) we averaged the folding (unfolding) rates obtained from each TDP peak/transition. How to cite this article : Chatterjee, S. et al. Mechanistic insight into the interaction of BLM helicase with intra-strand G-quadruplex structures. Nat. Commun. 5:5556 doi: 10.1038/ncomms6556 (2014).